Remodelling of a homeobox gene cluster by multiple independent gene reunions inDrosophila Genome clustering of homeobox genes is often thought to reflect arrangements of tandem gene duplicates maintained by advantageous coordinated gene regulation. Here we analyse the chromosomal organization of the NK homeobox genes, presumed to be part of a single cluster in the Bilaterian ancestor, across 20 arthropods. We find that the ProtoNK cluster was extensively fragmented in some lineages, showing that NK clustering in Drosophila species does not reflect selectively maintained gene arrangements. More importantly, the arrangement of NK and neighbouring genes across the phylogeny supports that, in two instances within the Drosophila genus, some cluster remnants became reunited via large-scale chromosomal rearrangements. Simulated scenarios of chromosome evolution indicate that these reunion events are unlikely unless the genome neighbourhoods harbouring the participating genes tend to colocalize in the nucleus. Our results underscore how mechanisms other than tandem gene duplication can result in paralogous gene clustering during genome evolution. Clusters of paralogous genes are thought to result predominantly from tandem gene duplications [1] . Paralogues within these clusters are functionally related, playing pivotal roles for the organism, such as oxygen transport (globin genes [2] , [3] ) and development (Hox genes [4] ). To date, analysis of the varying degree of Hox gene clustering across taxa has been instrumental for understanding the interface between the evolution, function and organization of paralogous gene clusters in animal genomes [5] . Thus, the evolutionary conservation of the ancient clustering of Hox genes in vertebrate lineages is thought to reflect a constraint imposed by the sequential expression of these genes during development, which parallels how they are ordered in the cluster [5] , [6] . The mechanistic bases underlying this temporal collinearity are not fully understood, but are consistent with a delicate, coordinated regulation of the constituent genes [7] , [8] . Importantly, species lacking these developmental constraints exhibit a more fragmented organization of the Hox cluster [5] , [9] , as illustrated by the genus Drosophila [10] . This notion of coordinated gene expression regulation being linked to the organization of clustered paralogous genes has been posited for other paralogous gene clusters, including the NK cluster in D. melanogaster [11] , [12] . NK genes are an important class of homeobox genes that dictate mesoderm development in Bilateria [12] , [13] , [14] . Unlike the Hox genes, extended clustering of NK genes is found in insect species, which contrasts with their dispersion in vertebrates [13] , [15] . Further identification of NK cluster conservation in additional genomes, especially in those known to be highly rearranged, would reinforce the notion that the conservation of the NK cluster in some taxa is because of functional requirements. However, this hypothesis remains unexplored. Another poorly understood structural aspect of the genomic arrangement of the NK genes is the subtle differences in NK cluster composition among the arthropods characterized to date. Genome mapping information from deuterostome and protostome species supports the existence of a ProtoNK cluster consisting of nine genes: Msx , NK4 , NK3 , Lbx , Tlx , NK7 , NK6 , NK1 and NK5 (refs 13 , 16 , 17 , 18 ). Regardless of some lineage-specific duplications, clusters of five to six different NK genes containing the same set of four ( NK4 , NK3 , Lbx and Tlx ) are observed in Tribolium castaneum, Anopheles gambiae and D. melanogaster [12] , [13] , [15] . The presence of Msx in the cluster of the first two species and NK1 in that of D. melanogaster suggests important differences in how the ProtoNK cluster has been reshaped by structural variation during insect evolution. The increasing availability of insect genomes with limited assembly fragmentation now allows for an accurate examination of lineage-specific evolutionary patterns that can be highly informative about the features that are essential to the genome organization of NK genes. Here we performed a comprehensive analysis of the organization of the nine NK genes belonging to the putative ProtoNK cluster and their neighbouring genes. This was performed across 20 arthropods in order to: (i) ascertain the extent of conservation of NK clustering when multiple highly rearranged genomes, such as those in the Drosophila genus and Culicidae, are considered [19] , [20] , [21] ; (ii) understand the origin of differences in constituent genes that NK clusters show among different arthropod phyla by reconstructing the evolutionary history of NK gene rearrangements; and (iii) extract evolutionary patterns of how the organization of a paralogous gene cluster decays and is reshaped in animal genomes. We find compelling evidence of a more malleable chromosomal organization of NK genes than previously noted in insects, which conflicts with the notion of clustering conservation due to regulatory-based constraints. Importantly, the reconstruction of the evolutionary history of the ProtoNK cluster in arthropods, and the analyses of gene neighbourhoods, unveil two independent reunions of previously separated NK genes during the evolution of the genus Drosophila . Simulation of chromosome evolution under different scenarios point to a nonrandom mode of evolution that requires a facilitation process. The evolution of the NK cluster highlights how neglected evolutionary processes, as a result of their apparent improbability, may have played a critical role in reshaping paralogous gene clustering in animal genomes. Mapping and annotating NK genes in Arthropoda We performed genome mapping and revised the annotations of NK genes in 17 Bilateria: 10 Drosophila species; three mosquito species; the silkworm; two Hymenoptera; and the crustacean Daphnia pulex (Methods; Supplementary Fig. 1 and Supplementary Data 1 ). The accuracy of our orthologous searches was ascertained by phylogenetic analysis of the homeodomain sequences ( Supplementary Figs 2 and 3 ). Together with comparative genome data comprising an additional six Bilateria including D. melanogaster , An. gambiae , the red flour beetle, the ragworm, the lancelet and humans [13] , [15] , [18] , [22] , [23] , we laid out the organization of NK genes within the ProtoNK cluster ( Fig. 1 ). Contiguities between NK genes among deuterostomes and protostomes were in good agreement, with the exception of the downstream neighbour to Tlx. In the lancelet, NK7, and not NK1 ( slou ) as in D. melanogaster , is downstream of Tlx. Evolutionary stability of the lancelet genome at the structural level compared with other deuterostome [24] , [25] and some protostome lineages, such as those of Diptera [26] , [27] , point to Tlx–NK7 as the most likely ancestral contiguity in the Bilaterian common ancestor. Further, and unlike in other reconstructions of the NK gene organization in this ancestor [13] , [15] , [23] , NK1 was inferred to be adjacent to Msx because of their proximity (~76 kb and three intervening genes) within the scaffold 186 of the D. pulex assembly ( Supplementary Data 1 and 2 ). 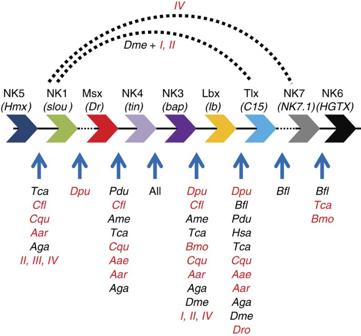Figure 1: Supported contiguities between nine NK genes in the ProtoNK cluster across Bilateria. Contiguities denoting close physical proximity in at least one deuterostome and one protostome species (subtaxa of the Bilateria) are indicated by a solid line between genes. Dotted lines indicate contiguities denoting close physical proximity only in deuterostome or protostome species. Species:Pdu, Platynereis dumerilii; Bfl,Branchiostoma floridae;Hsa, Homo sapiens; Dpu, Daphnia pulex; Cfl, Camponotus floridanus; Ame, Apis mellifera; Tca, Tribolium castaneum; Bmo, Bombyx mori; Cqu, Culex quinquefasciatus; Aae, Aedes aegypty; Aga, Anopheles gambiae; Aar, Anopheles arabiensis; Dme, D. melanogaster(refs12,13,15,18,23,33, black; this work, red).Dro, allDrosophilaspecies exceptD. melanogaster.I–IV,Drosophilaspecies showing different organization modes for NK genes. Gene names inD. melanogasterare indicated in parenthesis. Contiguity of NK genes was inferred forP. dumeriliibased on proximity ofin situhybridization signals from different genes18. Figure 1: Supported contiguities between nine NK genes in the ProtoNK cluster across Bilateria. Contiguities denoting close physical proximity in at least one deuterostome and one protostome species (subtaxa of the Bilateria) are indicated by a solid line between genes. Dotted lines indicate contiguities denoting close physical proximity only in deuterostome or protostome species. Species: Pdu, Platynereis dumerilii; Bfl , Branchiostoma floridae ; Hsa, Homo sapiens; Dpu, Daphnia pulex; Cfl, Camponotus floridanus; Ame, Apis mellifera; Tca, Tribolium castaneum; Bmo, Bombyx mori; Cqu, Culex quinquefasciatus; Aae, Aedes aegypty; Aga, Anopheles gambiae; Aar, Anopheles arabiensis; Dme, D. melanogaster (refs 12 , 13 , 15 , 18 , 23 , 33 , black; this work, red). Dro , all Drosophila species except D. melanogaster . I–IV , Drosophila species showing different organization modes for NK genes. Gene names in D. melanogaster are indicated in parenthesis. Contiguity of NK genes was inferred for P. dumerilii based on proximity of in situ hybridization signals from different genes [18] . Full size image A malleable NK gene cluster in the genus Drosophila Next, we tested the consistency of the extended NK clustering by examining the structurally dynamic genome of Drosophila species [26] , [27] . We determined which chromosomal regions with conserved local gene order, that is, microsynteny blocks, among the 2,683 delineated across nine Drosophila species [27] harbour at least one NK gene. These species accumulate a total divergence time of ~380 million years and represent the two main subgenera of the genus Drosophila [28] . NK genes were located in seven microsynteny blocks ( Fig. 2 ; Supplementary Data 3 ) that are part of two of the five rod-like chromosomes that form the Drosophila karyotype (Muller’s elements D and E [29] ). Importantly, genes clustered at cytological position 3R (93DE) of D. melanogaster ( tin, bap, lbe/lbl, C15 and slou ) [12] , [30] were found scattered over three microsynteny blocks ( Fig. 2 , shaded in salmon), which are separated by long chromosomal distances in species from both the Drosophila and Sophophora subgenera. 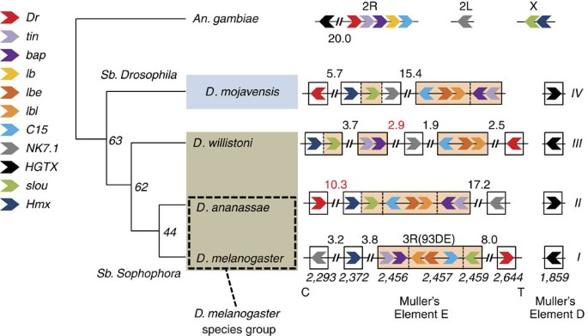Figure 2: Four different chromosomal organization modes of NK genes in the genusDrosophila. The organization of NK genes in a different Diptera lineage is included as an outgroup. Lbx is duplicated (lb, lbeandlbl) in allDrosophilaspecies (ref.12and this work). Gene order and orientation were obtained from previous reconstructions of local gene order in theDrosophilagenus27andAn. gambiae13,15, plus existing gene annotations or revisions of these. Only one species from each organization mode in the genusDrosophilais shown. Note that, although only NK genes are shown, these genes are in most cases part of microsynteny blocks where other genes reside. The identifiers of these microsynteny blocks according to (ref.27) are indicated below their arrangement inD. melanogaster. Only the microsynteny block harbouringHGTXis located on Muller’s chromosomal element D; the rest reside in Muller’s chromosomal element E. Microsynteny blocks located at the cytological location3R(93DE) ofD. melanogasterare shown in salmon. Double forward slash: molecular discontinuities between consecutive NK genes. The approximate distance in Mb is indicated; estimates obtained on merging appropriate scaffolds using gene order information as a guide are shown in red. For theDrosophilaMuller’s element E only: C, centromere; T, telomere. The phylogenetic relationships among species are as described28,57, and the estimated divergence times are indicated in millions of years28. Species belonging to the two main subgenera of the genusDrosophila, DrosophilaandSophophora, are squared in purple and brown, respectively. Branch length not to scale. Figure 2: Four different chromosomal organization modes of NK genes in the genus Drosophila . The organization of NK genes in a different Diptera lineage is included as an outgroup. Lbx is duplicated ( lb, lbe and lbl ) in all Drosophila species (ref. 12 and this work). Gene order and orientation were obtained from previous reconstructions of local gene order in the Drosophila genus [27] and An. gambiae [13] , [15] , plus existing gene annotations or revisions of these. Only one species from each organization mode in the genus Drosophila is shown. Note that, although only NK genes are shown, these genes are in most cases part of microsynteny blocks where other genes reside. The identifiers of these microsynteny blocks according to (ref. 27 ) are indicated below their arrangement in D. melanogaster . Only the microsynteny block harbouring HGTX is located on Muller’s chromosomal element D; the rest reside in Muller’s chromosomal element E. Microsynteny blocks located at the cytological location 3R (93DE) of D. melanogaster are shown in salmon. Double forward slash: molecular discontinuities between consecutive NK genes. The approximate distance in Mb is indicated; estimates obtained on merging appropriate scaffolds using gene order information as a guide are shown in red. For the Drosophila Muller’s element E only: C, centromere; T, telomere. The phylogenetic relationships among species are as described [28] , [57] , and the estimated divergence times are indicated in millions of years [28] . Species belonging to the two main subgenera of the genus Drosophila, Drosophila and Sophophora , are squared in purple and brown, respectively. Branch length not to scale. Full size image Subsequently, we determined the precise chromosomal organization of NK genes in 11 Drosophila species using previously reconstructed gene orders [27] and existing information in FlyBase [31] . NK genes exhibited four organization modes along Muller’s element E in different lineages ( I–IV ; Fig. 2 ; Supplementary Fig. 1 ). To discard in silico errors in prior genome assembly reconstructions that could affect the chromosomal arrangement of NK genes, we mapped those genes located on the Muller’s element E using in situ hybridization on polytene chromosomes. We did so in species representative of the organization modes II ( D. ananassae ), III ( D willistoni ) and IV ( D. mojavensis ), finding full support to the chromosomal arrangements inferred in silico ( Supplementary Fig. 4 ). The dispersion pattern exhibited by the NK genes that form the D. melanogaster 93DE cluster in several lineages of the genus Drosophila clearly conflicts with the previous notion of regulatory-based constraints underlying cluster integrity [11] , [13] , [15] . In addition, the different organization modes helped identify the two NK gene contiguities ( tin-bap and lbe/lbl-C15 ) most likely to be under functional constraints in the genus Drosophila [22] ; these two contiguities are also conserved across 11 major metazoan lineages [32] . Overall, these results show no evidence for the ProtoNK cluster to have a markedly differential capacity to accommodate chromosomal splits between insect and vertebrate genomes during their evolution [13] , [15] . The genus Drosophila harbours unique NK gene contiguities To better understand the repatterning of NK genes that has led to their existing organization modes in the genus Drosophila , we used microsynteny information from this genus, eight additional holometabolous insects and the crustacean D. pulex ( Supplementary Fig. 1 ). The NK gene organization in D. melanogaster (mode I ) is only observed in its close relatives within the D. melanogaster subgroup; all these species shared a common ancestor 12.8 mya (ref. 28 ). D. ananassae (organization mode II ) exhibited a similar arrangement to that of species of organization mode I , but with the presence of Hmx immediately upstream of slou , which gives rise to the most extensive NK gene cluster among Bilateria. The contiguity between Hmx and slou is also seen in species with organization modes III and IV , three mosquito species, T. castaneum , and C. floridanus , pointing to an ancestral contiguity (refs 13 , 33 and this work) that must have been disrupted after divergence of the D. ananassae and D. melanogaster lineages. Further, the species displaying the organization mode III showed the most disintegrated configuration of NK genes, involving two novel discontiguities relative to organization modes I and II : one between bap and lbe/lbl and the other between slou and C15 . The discontiguity between bap and lbe/lbl is only additionally observed in Aedes aegypti , and therefore represents the result of a recent split, which must have happened independently in several lineages within organization mode III on the basis of the currently accepted phylogeny [28] ( Supplementary Fig. 1 ). In contrast, the discontiguity between slou and C15 is the norm in other arthropods ( Fig. 1 and Supplementary Fig. 1 ). Lastly, the three species of the subgenus Drosophila displayed organization mode IV , which includes the discontiguity between slou and C15 , plus an unexpected close proximity between NK7.1 and the gene pair slou–Hmx . The gene Dr is not clustered with any other NK genes in all Drosophila species, which combined with its contiguity to tin in Hymenoptera, T. castaneum and mosquitoes, suggests that Dr dissociation from tin occurred in a recent common ancestor to the Drosophila and Sophophora subgenera. Beyond helping to reconstruct the sequence of chromosomal rearrangements that have influenced the organization of NK genes in insects, this comparative analysis uncovers two contiguities between NK genes that are unique among Bilateria. Unique contiguities between NK genes are secondarily derived What evolutionary scenarios can explain the contiguities of C15 and slou in the species with organization modes I and II , and that of NK7.1 and slou in the species with organization mode IV ? One scenario assumes that such contiguities reflect ancestral gene associations in insects, only remaining undisrupted in particular lineages. A second scenario proposes that the arrangement of the NK genes has been reshaped mostly by small-scale rearrangements, with the focal NK genes always remaining in close proximity in the same chromosomal region, and irrespective of the lineage. Eventually, additional small-scale rearrangements, for example, microinversions, would juxtapose the focal NK genes as they appear in particular contemporary species. In contrast, in the remaining lineages, this close proximity would be disrupted via large-scale rearrangements. Lastly, a third scenario postulates that any close proximity between the focal NK genes would have been initially altered and later re-established in unusual arrangements by large-scale rearrangements. The first scenario can be ruled out since such contiguities involve C15 and NK7.1 downstream of the same gene, slou , and both contiguities ( C15–slou and NK7.1–slou ) could not be present simultaneously in the Bilaterian ancestor, that is, they are mutually exclusive. The second scenario also faces insurmountable difficulties ( Supplementary Fig. 5a,b ). First, a close proximity between focal NK genes can only be maintained if the chromosomal region where they reside escapes from, or is refractory to, the chromosomal rearrangements that have reshaped the Drosophila genome. This is specially unlikely considering the thousands of paracentric inversions estimated to have occurred [26] , [27] , and the lack of evidence for extended functional constraints keeping most NK genes together. Second, analyses of gene neighbourhoods within and outside of the genus Drosophila show that several NK genes, including C15 and NK7.1 , were certainly flanked by multiple non-NK genes in the ancestor to the genus Drosophila ; this conflicts with any presumed evolutionarily maintained proximity among the focal NK genes ( Supplementary Figs 5a,b and 6 ; Supplementary Note 1 ). These contiguities between NK and non-NK genes have remained until present times in the form of tight associations that can be tracked throughout the genus Drosophila ( Supplementary Data 3 ). In addition, conflicting with a presumed maintained proximity, the possible arrangements of the focal NK genes in the ancestor to the genus Drosophila show the mutually exclusive nature of both contiguities, such that one of them can only be originated if the focal NK genes were distantly located. Moreover, third, numerous ad hoc rearrangements have to be postulated in order to recreate the arrangement of the focal NK genes in the ancestor to the genus Drosophila that is compatible with the information provided by the analysis of gene neighbourhoods. These rearrangements include microinversions and conservative gene transpositions, which are known to occur at a very low frequency in the genus Drosophila ( Supplementary Note 1 ). All these difficulties do not apply to the scenario that postulates the eventual reunion events ( Supplementary Figs 5c,7 and 8 ). Consistent with gene neighbourhood information, some focal NK genes would be flanked by multiple non-NK genes, being separated from each other by long chromosomal distances in the ancestor to the genus Drosophila . This lack of close proximity necessarily implies the occurrence of large-scale rearrangements resulting in the unique contiguities seen in particular contemporary species. In addition, this scenario postulates a lower number of ad hoc rearrangements and does not include small-scale rearrangements ( Fig. 3 ). Collectively, the contrasting plausibility of these three scenarios strongly suggests that the contiguities between C15 and slou in species with organization modes I and II , and that between NK7.1 and slou in species with organization mode IV are secondarily derived. 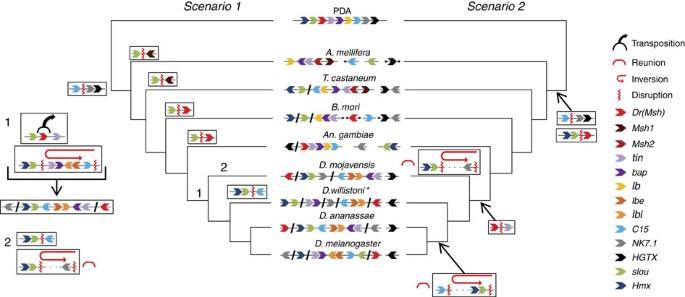Figure 3: Evolutionary scenarios explaining the contiguity betweenC15andslouinD. melanogasterandD. ananassae. Left; scenario 1 assumes that the contiguityC15–slouresulted from a microinversion that juxtaposed the focal genes, which were maintained in close proximity until theDrosophilagenus. In addition, an initial disruption (red wavy line) movedNK7.1andHGTXaway from the rest of the NK genes. In non-Drosophilalineages, repeated disruptions occurred betweenslouandDr. At the ancestor to theDrosophilagenus,Drwas transposed out along with its neighboursTrc8andCG2010, keeping the remaining NK genes in close proximity. Subsequently, a microinversion that includestin, bap, lbe, lblandC15led to theC15–sloucontiguity seen in contemporary species with organization modesIandII. This contiguity was broken in the lineages leading to species with organization modesIIIandIV; twice independently in organization modeIIIaccording to the current phylogeny ofDrosophila28. Right; scenario 2 assumes that theC15–sloucontiguity was the by-product (asterisk) of a large-scale rearrangement after the radiation of the genusDrosophila. In this scenario,C15andslouwere not in close proximity, at least in the ancestor to the genusDrosophila. The reunion of these genes would have occurred after the lineage that leads to the species with organization modesIandIIbranched off from the lineage leading to the species with organization modeIII. In addition, two initial chromosomal rearrangements separatedNK7.1–HGTXandslou–Hmxfrom the rest of the ProtoNK cluster. Regardless of the scenario, the contiguity betweenNK7.1andslou–Hmxmust result from a large-scale rearrangement in the lineage leading to species with organization modeIV. In total, 11 and 5 rearrangements are postulated in scenarios 1 and 2, respectively. A variant of the scenario 1 is possible but involves 17 rearrangements. Forward slash: molecular discontinuity. Terminal diamond: uncertain molecular discontinuities associated with assembly fragmentation. PDA: protostome–deuterostome ancestor. Figure 3: Evolutionary scenarios explaining the contiguity between C15 and slou in D. melanogaster and D. ananassae . Left; scenario 1 assumes that the contiguity C15–slou resulted from a microinversion that juxtaposed the focal genes, which were maintained in close proximity until the Drosophila genus. In addition, an initial disruption (red wavy line) moved NK7.1 and HGTX away from the rest of the NK genes. In non- Drosophila lineages, repeated disruptions occurred between slou and Dr . At the ancestor to the Drosophila genus, Dr was transposed out along with its neighbours Trc8 and CG2010 , keeping the remaining NK genes in close proximity. Subsequently, a microinversion that includes tin, bap, lbe, lbl and C15 led to the C15–slou contiguity seen in contemporary species with organization modes I and II . This contiguity was broken in the lineages leading to species with organization modes III and IV ; twice independently in organization mode III according to the current phylogeny of Drosophila [28] . Right; scenario 2 assumes that the C15–slou contiguity was the by-product (asterisk) of a large-scale rearrangement after the radiation of the genus Drosophila . In this scenario, C15 and slou were not in close proximity, at least in the ancestor to the genus Drosophila . The reunion of these genes would have occurred after the lineage that leads to the species with organization modes I and II branched off from the lineage leading to the species with organization mode III . In addition, two initial chromosomal rearrangements separated NK7.1–HGTX and slou–Hmx from the rest of the ProtoNK cluster. Regardless of the scenario, the contiguity between NK7.1 and slou–Hmx must result from a large-scale rearrangement in the lineage leading to species with organization mode IV . In total, 11 and 5 rearrangements are postulated in scenarios 1 and 2, respectively. A variant of the scenario 1 is possible but involves 17 rearrangements. Forward slash: molecular discontinuity. Terminal diamond: uncertain molecular discontinuities associated with assembly fragmentation. PDA: protostome–deuterostome ancestor. Full size image Large chromosomal rearrangements can mediate gene reunions How often do genes from the same ancestral cluster become separated and then reunited again via large chromosome repatterning during evolution? At least, two other cases are reminiscent of the unique contiguities reported here, both involving homeobox genes. The first involves the Hox genes lab and abd-A , which belong to the Antennapedia and Bithorax homeotic complexes, respectively; their reunion would have taken place in the lineage that leads to the D. repleta species group [34] . The second case involves the relocation of a Hox gene, which was moved to a different chromosome next to two NK genes in the lineage of P. dumerilii [18] . Nevertheless, it is unclear whether this kind of reunion event can occur passively as a mere by-product of the magnitude and mode of chromosome repatterning. Knowing that the gene arrangement of the Muller’s chromosomal element E has been reshaped mostly by 614 chromosomal paracentric inversions in the genus Drosophila [27] , we mimicked the evolution of this chromosome in silico and determined how often separated microsynteny blocks become reunited. To illustrate this process, we focused on the microsynteny blocks containing C15 and slou and used their arrangement in D. mojavensis (separated) and in D. melanogaster (adjacent) as starting and finishing points, respectively ( Supplementary Note 2 ). We performed this analysis considering several magnitudes of chromosome repatterning, different degrees of proximity between the focal microsynteny blocks and different dynamics on how inversion breakpoints occur—either at random or alternatively reflecting previously estimated levels of local fragility [27] ( Fig. 4a,b ). In all cases, the probability of a reunion event was <0.05. This conclusion held when the analysis was repeated with a different starting ( D. willistoni ) or final ( D. ananassae ) genome ( Supplementary Table 2 ). Subsequently, we implemented additional conditions including a selective advantage, for example, facilitated co-regulation, once a serendipitous contiguity of NK genes occurred. Only in one of the tested scenarios, under the most favourable set of conditions, was it possible to observe the reunion of C15 and slou at P~ 0.07. Taken together, a passive chromosomal rearrangement process has a very low probability of mediating the reunion of NK genes regardless of how chromosomal rearrangements become generated and the adaptive value the contiguity between NK genes confers to the carriers once it is established. 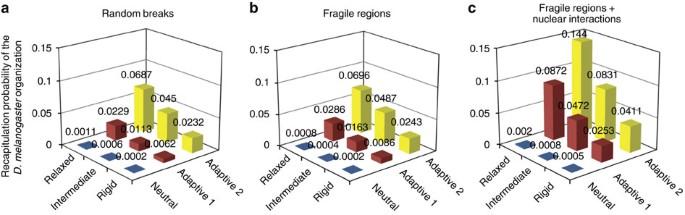Figure 4: Simulation results showing the probability of a chromosomal rearrangement-mediated reunion of microsynteny blocks harbouringC15andslou. The simulations start from the microsynteny block arrangement inD. mojavensisand then proceed by accumulating chromosomal inversions. The number of inversions simulated was 10 times the minimum estimate calculated to differentiate the genomes ofD. mojavensisandD. melanogasterunder maximum parsimony27. At the end of each simulation, whether the observed microsynteny block arrangement inD. melanogasterwas achieved is determined, and the number of times this recapitulation occurs recorded and expressed as a fraction of total number of simulations performed (10,000). Results show when inversion breakpoints are assumed to occur at random (a), reflecting previously estimated variable levels of fragility across microsynteny blocks27(b), and likebbut the chromosomal inversion rate between microsynteny blocks harbouring NK genes being increased because of prior physical proximity in the nucleus (c). The recapitulation of the organization inD. melanogasterwas examined while varying several parameters. The first (xaxis) is how well properties such as orientation and relative order of microsynteny blocks harbouring NK genes resemble the observed configuration inD. melanogaster. The clustering levels analysed are:rigid, identical relative microsynteny block order and orientation to the target genome;intermediate, identical relative microsynteny block order to the target genome regardless of the orientation; relaxed, physical proximity regardless of the order and orientation. The second parameter (zaxis) is the adaptive impact that such clustering represents, ranging from none (neutral;once clustering is achieved it can be disrupted again by a subsequent chromosomal inversion) to an advantageous effect, for example, because of co-regulation, which results in protecting the contiguity between microsynteny blocks carrying the NK genes from being disrupted by subsequent rearrangements. This advantageous effect is mimicked at varying distances between the NK genes involved. Inadaptive 1, no intermingled microsynteny block is allowed between those harbouring NK genes. Inadaptive 2, one microsynteny block, regardless of its size, is allowed. Figure 4: Simulation results showing the probability of a chromosomal rearrangement-mediated reunion of microsynteny blocks harbouring C15 and slou . The simulations start from the microsynteny block arrangement in D. mojavensis and then proceed by accumulating chromosomal inversions. The number of inversions simulated was 10 times the minimum estimate calculated to differentiate the genomes of D. mojavensis and D. melanogaster under maximum parsimony [27] . At the end of each simulation, whether the observed microsynteny block arrangement in D. melanogaster was achieved is determined, and the number of times this recapitulation occurs recorded and expressed as a fraction of total number of simulations performed (10,000). Results show when inversion breakpoints are assumed to occur at random ( a ), reflecting previously estimated variable levels of fragility across microsynteny blocks [27] ( b ), and like b but the chromosomal inversion rate between microsynteny blocks harbouring NK genes being increased because of prior physical proximity in the nucleus ( c ). The recapitulation of the organization in D. melanogaster was examined while varying several parameters. The first ( x axis) is how well properties such as orientation and relative order of microsynteny blocks harbouring NK genes resemble the observed configuration in D. melanogaster . The clustering levels analysed are: rigid , identical relative microsynteny block order and orientation to the target genome; intermediate , identical relative microsynteny block order to the target genome regardless of the orientation ; relaxed , physical proximity regardless of the order and orientation. The second parameter ( z axis) is the adaptive impact that such clustering represents, ranging from none ( neutral; once clustering is achieved it can be disrupted again by a subsequent chromosomal inversion) to an advantageous effect, for example, because of co-regulation, which results in protecting the contiguity between microsynteny blocks carrying the NK genes from being disrupted by subsequent rearrangements. This advantageous effect is mimicked at varying distances between the NK genes involved. In adaptive 1 , no intermingled microsynteny block is allowed between those harbouring NK genes. In adaptive 2 , one microsynteny block, regardless of its size, is allowed. Full size image Large-scale chromosomal rearrangements reshape gene organization over evolutionary time. This occurs by disrupting existing gene neighbourhoods and creating new ones. Our analysis on the gene organization of NK genes in insects revealed several gene contiguities that are fully consistent with a evolutionary-derived origin in independent lineages of the genus Drosophila . These contiguities would be the by-product of large-scale chromosomal inversions. Nevertheless, simulated evolutionary scenarios indicate that a passive chromosome evolutionary mode does not suffice to explain the reunions of NK genes. Additional factors or mechanisms might increase this probability, especially when functionally related genes are involved. For example, the relocation of lab in the D. repleta species group [34] , [35] has been suggested to result from a rearrangement upon the nuclear colocalization of separated genome neighbourhoods harbouring Hox genes [36] . Specifically, genes from the Antennapedia and Bithorax complexes have been shown to be spatially close to each other during their repression by Polycomb protein complexes in some tissues. Importantly, one of the 268 significant contacts between genome neighbourhoods identified in D. melanogaster embryos involved two Polycomb domains harbouring slou and other NK genes, such as the lady bird genes [37] . We propose that similar scenarios of coordinated repression or activation, accompanied by nuclear colocalization in the germline, brought different NK-harbouring genome neighbourhoods together more often than those same neighbourhoods are brought together with others without coordinated regulation. This recurrent physical proximity, if coupled with chromosomal breaks and illegitimate end-joining, results in an increased probability of chromosomal rearrangement between functionally related genome neighbourhoods, which would lead to the reunion of remnants of a previously disrupted ProtoNK cluster. When this mechanism is implemented in chromosome evolution simulations, the probability of recapitulating the organization of NK genes observed in D. melanogaster increases up to P =0.14, using D. mojavensis as a starting genome ( Fig. 4c ; Supplementary Table 2 ). An important underlying supposition to this cascade of events is that nuclear colocalization among functionally related genes must be conserved across distantly related lineages. This has been demonstrated in mammals, yeast and for the Hox genes between the distantly related species D. melanogaster and D. virilis [36] , [38] , [39] . A tantalizing prediction within this model of frequent nuclear colocalization events, coupled with recurrent chromosome rearrangements that facilitate reunions, is that it should affect both NK and non-NK genes present in the same genome neighbourhoods. To test this hypothesis, we analysed the location of genes in microsynteny blocks adjacent to those harbouring NK genes across the genus Drosophila and other arthropods. In three instances ( Crz , CG2321 and CG16791 ; Supplementary Figs 9–11 ), the same non-NK gene was found to flank different NK genes in different lineages, thus suggesting that this nonrandom pattern of gene reorganization operates on a global scale in the genome neighbourhoods where the NK genes reside but not specifically on these genes. Nonparalogous but functionally related genes have been shown to cluster in the genome upon relocation via chromosomal rearrangements both in plants [40] and fungi [41] , [42] . In the case of paralogous genes, genome clustering is assumed to result from tandem duplication events. The unique contiguities between NK genes documented here support that paralogous gene clustering can also be secondarily originated via large-scale chromosomal rearrangements. Whether the proposed model of reiterated involvement of the same genome neighbourhoods in chromosomal rearrangements, and its effect on the composition of the NK and Hox gene clusters, applies to other eukaryotic clusters of paralogous genes remains to be established. Genome mapping and annotation of NK genes For Drosophila species other than D. melanogaster , locations of NK genes were extracted from reconstructed gene orders [27] and from FlyBase when annotated. In the absence of orthologue calls, we used D. melanogaster transcript and protein sequences of NK genes in BLASTn and tBLASTn reciprocal best hit searches [43] , [44] , [45] . For non- Drosophila species, we proceeded likewise using appropriate genome databases ( Supplementary Data 1 ) and, in the absence of any annotation, we used An. gambiae and T. castaneum as reference species for locating and annotating NK genes in mosquitoes and non-Diptera species, respectively. All previous annotations were evaluated and refined when necessary ( Supplementary Data 1 ). The existence of a molecular discontinuity between consecutive NK genes on the same chromosome, or scaffold, was established in two different ways: for Drosophila species, when more than one microsynteny block separated those harbouring the NK genes; for non- Drosophila species, when the number of intervening annotated genes was more than four and the distance expressed as a fraction of the genome size of the species in question was >0.1% ( Supplementary Data 2 ). Phylogenetic analysis Amino-acid sequences of the homeodomain of NK genes were obtained from the database HomeoDB 2 (refs 46 , 47 ) and our own reannotation. The evolutionary history of the sequences was inferred using maximum likelihood and neighbour-joining methods based on the JTT model of amino-acid substitutions [48] , [49] , [50] . For maximum likelihood, a discrete Gamma distribution was used to model evolutionary rate differences among sites (five categories; + G , parameter=0.4000). For neighbour-joining, the rate of variation among sites was modelled with a gamma distribution (shape parameter=1). The analysis involved 190 amino-acid sequences; all ambiguous positions were removed for each sequence pair. Bootstrapping (1,000 replicates) was performed to determine the confidence of the branches. With the exception of sequence retrieval, all other steps were conducted in MEGA 6.0 (ref. 51 ). Aligned sequences are provided in Supplementary Fig. 2 . Strains Previously sequenced stocks [52] were obtained from the UC San Diego Drosophila Stock Center: D. ananassae (14024-0371.13), D. mojavensis (15081-1352.22) and D. willistoni (14030-0811.24). In situ hybridization experiments Species-specific probes were designed for NK genes on Muller's element E; only one of the two tandemly duplicated Lbx genes, lbe , was mapped. Gene sequences were retrieved from FlyBase when the orthologue of the gene in D. melanogaster was available. Otherwise, the orthologue was annotated as described above. Primer 3 was used for primer design [53] . Takara Ex Taq and Takara Taq, depending on the size of the fragment to be amplified, were used following manufacturer’s conditions. Supplementary Table 1 shows primers and PCR amplification conditions used. Genomic DNA was extracted using the DNeasy Blood & Tissue kit (Qiagen). The TOPO TA Cloning Kit for Sequencing (Life Technologies) was used to clone desired PCR fragments. All the cloned fragments were verified by Sanger sequencing and subsequent BLASTn analysis [44] . Salivary gland chromosome preparation, hybridization and probe detection were carried out for all species according to standard procedures [54] . Probe labelling by nick translation was carried out using the Biotin Nick Translation Mix (Roche). Micrographs were taken with a Nikon Eclipse 90i-automated microscope under phase contrast. Hybridization signal localization was carried out using available photomaps of D. ananassae, D. mojavensis and D. willistoni [55] . Data sets Comparative microsynteny maps in the genus Drosophila were obtained from ref. 27 ; the type of maps used included the requirement of conservation of gene order but not orientation (GO synteny definition). The differential probability of microsynteny blocks to locate at the edge of a chromosomal inversion, that is, the estimates of local fragility across the genome, were taken also from ref. 27 . In silico chromosome evolution A chromosome-mimicking Muller's element E in microsynteny block composition and orientation was recreated based on [27] . This initial chromosome was different depending on the evolutionary scenario analysed. Three different types of scenarios were simulated: (i) between D. mojavensis and D. melanogaster; (ii) between D. willistoni and D. melanogaster; and (iii) between D. mojavensis and D. ananassae . A particular number of inversions, n , which was previously obtained using MGR [27] , [56] , or n × 10, was applied to the initial chromosome of each scenario, which resulted in the reshuffling of the constituent microsynteny blocks. For each type of scenario, 10,000 simulations were executed. In each simulation, whether the reunion of a particular set of microsynteny blocks including NK genes had occurred or not was examined. A range of conditions having an impact on the probability of this reunion was explored ( Supplementary Note 1 ). Code Accessibility The Python code used to implement the simulations is available as ( Supplementary Software 1 ). How to cite this article: Chan, C. et al . Remodelling of a homeobox gene cluster by multiple independent gene reunions in Drosophila . Nat. Commun . 6:6509 doi: 10.1038/ncomms7509 (2015).